Total synthesis of avenaol Avenaol, isolated from the allelopathic plant black oat, was the first C 20 germination stimulant related to strigolactones. Structurally, it consisted of a bicyclo[4.1.0]heptanone skeleton containing a cyclopropane ring bearing three main chains projecting in the same direction (i.e. all -cis- substituted cyclopropane). Herein, we report the total synthesis of avenaol using a robust strategy involving the formation of an all- cis -substituted cyclopropane via an alkylidenecyclopropane. The key factors in the success of this total synthesis include the Rh-catalysed intramolecular cyclopropanation of an allene, an Ir-catalysed stereoselective double-bond isomerisation, and the differentiation of two hydroxymethyl groups via the regioselective formation and oxidation of a tetrahydropyran based on the reactivity of a cyclopropyl group. This strategy effectively avoids the undesired ring opening of the cyclopropane ring and the formation of a caged structure. Furthermore, this study confirms the proposed structure of avenaol, including its unique all- cis -substituted cyclopropane moiety. Natural products containing complex three-dimensional structures represent challenging synthetic targets, and compounds of this type have consequently received considerable interest from research groups all over the world [1] , [2] , [3] . Notably, cage-shaped natural products have been reported to show several interesting biological activities, and numerous polycyclic terpene [4] , [5] , [6] , [7] and alkaloid [8] targets of this type have inspired synthetic chemists to develop innovative new strategies to access these compounds. Non-cage-shaped natural products that are capable of being converted to cage-shaped materials also exhibit an interesting range of biological activities, as exemplified by avenaol [9] , shagene A [10] , erythrolide A [11] and arisanlactone C [12] (Fig. 1a ). These compounds are characterised by their bicyclo[4.1.0]heptane (avenaol, shagene A), bicyclo[3.1.0]hexane (erythrolide A), and bicyclo[6.1.0]nonane (arisanlactone C) skeletons, all of which contain a cyclopropane ring bearing three main chains projecting in the same direction (i.e. an all -cis- substituted cyclopropane). Although the synthesis of these natural products is considered to be as challenging as the synthesis of their cage-shaped counterparts, there have been very few reports to date pertaining to the synthesis of all -cis- substituted cyclopropanes. In fact, there have been no reports to date concerning the total synthesis of non-cage-shaped natural products containing an all- cis -substituted cyclopropane. Furthermore, it is envisaged that these syntheses would lead to the identification of several stereochemically interesting structures. With this in mind, we became interested in investigating the synthesis of natural products containing an all- cis -substituted cyclopropane using the non-typical strigolactone avenaol, which shows important biological activity, as a representative example. Fig. 1 Natural products containing all- cis -substituted cyclopropanes. a Various natural products containing an all- cis -substituted cyclopropane, all of which have been reported to show intriguing biological activities. b The structures of avenaol and two typical strigolactones. The major differences between these compounds include the AB ring carbon skeleton and the connectivity between the BC rings. The construction of the AB ring of avenaol represents a challenging problem Full size image Avenaol ( 1 ), which was first isolated from the allelopathic plant black oat ( Avena strigosa Schreb.) by Yoneyama and co-workers in 2014, was the first reported natural C 20 germination stimulant structurally related to strigolactones (SLs) [9] . Extensive NMR and high-resolution mass spectrometry analyses indicated that the structure of 1 consisted of a bicyclo[4.1.0]heptanone skeleton, a C ring lactone, four contiguous stereogenic centres and an all -cis- substituted cyclopropane. Although the all -cis- substituted cyclopropane ring in 1 might readily cyclise to form a caged structure via the formation of a C–C bond between the A and C rings, the analytic data for this compound were consistent with a non-cage structure (Fig. 1b ). Given that the structure of avenaol differs from those of typical SLs such as strigol and orobanchol, it was designated as a novel class of SL. Avenaol shows potent germination-stimulating activity for Phelipanche ramosa seeds, but much lower activities for Striga hermonthica and Orobanche minor . Although the biosynthetic pathways and target protein of a few typical SLs have recently been reported [13] , [14] , the biological properties of compound 1 have been poorly explored. Further study is therefore required to understand the relationship between the properties of avenaol and those of a few typical SLs. Although a variety of different strategies have been reported for the synthesis of typical SLs [15] , [16] , [17] , [18] , [19] , [20] , [21] , [22] , [23] , [24] , [25] , there have been no reports to date for the synthesis of avenaol. Herein, we report the total synthesis of avenaol based on a strategy for the construction of all- cis- substituted cyclopropanes using alkylidenecyclopropane as a key intermediate. The core structure is constructed through the Rh-catalysed intramolecular cyclopropanation of an allene, and an Ir-catalysed stereoselective double-bond isomerisation. This strategy effectively avoids the undesired ring opening of the cyclopropane ring and the formation of a caged structure. Furthermore, this study confirms the proposed structure of avenaol, including its unique all- cis -substituted cyclopropane moiety. Retrosynthetic analysis The main challenges associated with the synthesis of avenaol include the construction of a bicyclo[4.1.0]heptanone skeleton containing an all- cis -substituted cyclopropane, controlling the stereochemistry at the C8 position of the C ring, and the introduction of a C3 hydroxyl group on the A ring. The construction of bicyclo[4.1.0]heptanone skeletons has mainly been investigated in the context of constructing caged structures [26] , [27] , [28] . For non-caged structure, the direct synthesis of these systems has been limited to the 1,4-addition of a suitable anion of a trans -chloroallylphosphonamide [29] or Ir-catalysed or Rh-catalysed cis -selective cyclopropanation reactions [30] , [31] . However, preliminary work in our own group has shown that these methods are unsuitable for the synthesis of avenaol (Supplementary Fig. 1 ). Furthermore, cyclopropane rings bearing an electron-withdrawing group can readily undergo a ring-opening reaction [32] , [33] , [34] , further highlighting the difficulties of this approach. On the basis of these issues, we envisioned that the use of alkylidenecyclopropane [35] as an appropriate intermediate would avoid an unwanted ring-opening reaction and the formation of a caged structure. We also envisioned that avenaol could be obtained from 2 by the dihydroxylation of its convex face and the introduction of the D ring (Fig. 2 ). The C ring lactone could be constructed by the diastereoselective transformation of the diol based on the reactivity of the cyclopropyl group in 3 , which could be obtained by introduction of a hydroxymethyl group to the all- cis- substituted cyclopropane 4 . Compound 4 could be synthesised by the intramolecular cyclopropanation of allene 6 , which could be readily prepared from aldehyde 7 , followed by double-bond isomerisation of alkylidenecyclopropane 5 . The intramolecular cyclopropanation of an allene to form a six-membered carbocycle has not been reported, indicating that development work would be required to allow for the construction of the bicyclo[4.1.0]heptanone core. Fig. 2 Retrosynthesis of avenaol ( 1 ). Our strategy is characterised by the use of an alkylidenecyclopropane intermediate 5 , providing a robust route to the required all- cis -substituted cyclopropane, while avoiding the undesired ring opening of the cyclopropane ring and the formation of a caged structure. The numbering of the carbon atoms is consistent with that used for avenaol. PMB p -methoxybenzyl Full size image Construction of an all- cis -substituted cyclopropane Our synthesis began with the preparation of the cyclisation precursor 6 (Fig. 3 ). The treatment of known aldehyde 7 [36] with 2-(prop-2-yn-1-yloxy)tetrahydro- 2H -pyran and BnMe 3 NOH [37] , followed by methylation and acidic treatment gave 8 . The subsequent hydroalumination of 8 , followed by the treatment of the resulting intermediate with iodine gave 9 [38] , which was converted to carboxylic acid 10a via sequential protection as a triisopropylsilyl (TIPS) ether, hydroboration and oxidation by 9-azanoradamantane N -oxyl (nor-AZADO) [39] . The cyclisation precursor α-diazo-β-ketonitrile 6a was synthesised by sequential β-ketonitrile formation and diazo transfer reactions [40] . A similar sequence was used to prepare the benzyl-protected methyl diazoketone 6b . The α-diazo-β-ketoester 6c and ketonitrile 6d were also synthesised via 10b (Supplementary Fig. 2 ). Fig. 3 Synthesis of all- cis -substituted cyclopropane 4 . Conditions: a HC≡CCH 2 OTHP, BnMe 3 NOH, DMSO, 94%; b NaH, MeI, THF–DMPU; c pyridinium p -toluenesulfonate, MeOH, 92% (two steps); d LiAlH 4 then I 2 , Et 2 O, −78 °C, 83%; e TIPSCl, imidazole, DMF, 84%; f 9-BBN, then aq. NaOH, aq. H 2 O 2 , 71%; g nor-AZADO, DAIB, CH 2 Cl 2 –pH 7 buffer, 78%; h PivCl, i Pr 2 NEt, then MeOH, DMAP, 89%; i lithium bis(trimethylsilyl)amide, CH 3 CN, THF, −78 °C, 97%; j (imidazoyl)SO 2 N 3 , pyridine, CH 3 CN, 87%; k NaBH 4 , CeCl 3 , MeOH 95%, (dr 17:1); l PMBCl, NaH, NaI, THF, 0–50 °C, 97%; m diisobutylaluminium hydride, toluene–THF, −78 °C to rt; n NaBH 4 , MeOH, 0 °C, 76% (two steps); o I 2 , PPh 3 , imidazole, CH 2 Cl 2 , 0 °C; 84%, p NaBH 4 , DMSO, 80 °C, 76%; q TBAF, THF, 97%; r [Ir(cod)(pyr)PCy 3 ]BAr F , CH 2 Cl 2 , H 2 , 68% (dr 10:1). THP tetrahydropyranyl, DMPU N , N ′-dimethylpropylene urea, triisopropylsilyl, DAIB (diacetoxyiodo)benzene, DMAP 4-dimethylaminopyridine, BAr F (3,5-bisCF 3 C 6 H 3 ) 4 B − Full size image We subsequently investigated the formation of the alkylidenecyclopropane intermediates via the intramolecular cyclopropanation of allenes 6a – d using a Rh or Cu catalyst [41] . 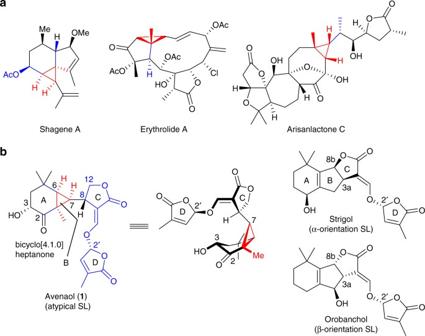Fig. 1 Natural products containing all-cis-substituted cyclopropanes.aVarious natural products containing an all-cis-substituted cyclopropane, all of which have been reported to show intriguing biological activities.bThe structures of avenaol and two typical strigolactones. The major differences between these compounds include the AB ring carbon skeleton and the connectivity between the BC rings. The construction of the AB ring of avenaol represents a challenging problem We initially investigated the cyclisation of methyl diazoketone 6b with Rh 2 (OAc) 4 , but this reaction failed to afford the desired cyclised product (Table 1 , entry 1). Substrates bearing a β-ketoester or ketonitrile instead of a methyl group were also evaluated in an attempt to stabilise the metal carbene. The reaction of 6c with Rh 2 (OAc) 4 or Cu(CH 3 CN) 4 PF 6 did not give the desired product (Table 1 , entries 2 and 3). In sharp contrast, the cyclisation reactions of the α-diazo-β-ketonitriles 6a and 6d with Rh 2 (OAc) 4 proceeded smoothly to give the alkylidenecyclopropanes 11a and 11d , respectively, in excellent yields, most likely because of the more electrophilic nature of the metal carbene (Table 1 , entries 4 and 5) [42] . It is noteworthy that this reaction only afforded the E isomer, because the metal carbene only approached from the less hindered face of the allene. For further transformation toward the all- cis -substituted cyclopropane, we used compound 11a because of the ease with which this compound could undergo protecting group manipulation. Table 1 Formation of alkylidenecyclopropane by allene cyclopropanation Full size table Next, we focused on the construction of the all- cis -substituted cyclopropane structure from alkylidenecyclopropane 11a . We initially investigated the hydrogenation of the alkylidenecyclopropanes (Supplementary Fig. 3 ). For example, compound 12 , which was prepared by reduction of 11a , followed by the PMB protection of the resulting alcohol, was hydrogenated over a Pd on carbon catalyst using H 2 gas. Surprisingly, this reaction gave the undesired trans isomer as the major product, most likely because of the steric effect of the nitrile group. We subsequently investigated the transition-metal-catalysed isomerisation of the double bond in this system using a directing group to reverse this selectivity. To determine the best position for the directing groups, we prepared alcohol 13 , silyl ether 14 and allyl alcohol 5 by the stepwise reduction of the nitrile group (Fig. 3 ). Despite our initial concerns regarding the ring-opening of the cyclopropane system during these transformations, the cyclopropane ring remained intact because it was stabilised as an alkylidenecyclopropane. 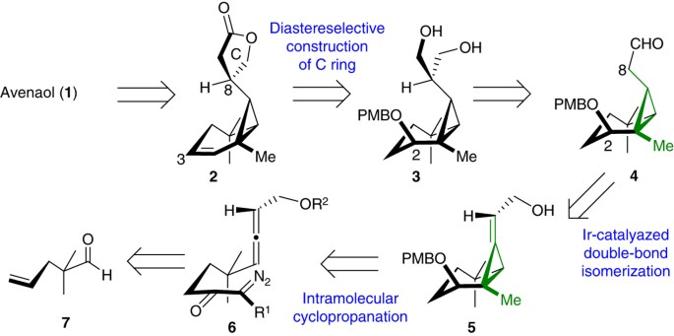Fig. 2 Retrosynthesis of avenaol (1). Our strategy is characterised by the use of an alkylidenecyclopropane intermediate5, providing a robust route to the required all-cis-substituted cyclopropane, while avoiding the undesired ring opening of the cyclopropane ring and the formation of a caged structure. The numbering of the carbon atoms is consistent with that used for avenaol. PMBp-methoxybenzyl Compound 12 was initially treated with Crabtree’s catalyst [43] , which was preactivated with H 2 , but failed to afford the all- cis -substituted cyclopropane (Table 2 , entry 1). Use of a substrate having nitrile and hydroxyl groups resulted in no reaction, and recovery of the starting material (Supplementary Fig. 4 ). These results indicated that the nitrile group deactivated the Ir catalyst rather than acting as a directing group. In contrast, the reaction of 13 bearing a hydroxymethyl group under these conditions, allowed for the successful isomerisation of the olefin under H 2 to give the silyl enol ether 15a in 92% yield with excellent stereoselectivity (Table 2 , entry 2). The success of this reaction indicated that the Ir catalyst approached from one face after its coordination to the alcohol (i.e. X , Fig. 4a ), resulting in the exclusive formation of the all- cis isomer. However, the hydroxymethyl group on 15a could not be converted to a methyl group without opening the cyclopropane ring. Notably, the treatment of silyl ether 14 with Crabtree’s catalyst resulted in very little reaction, because of the lack of a directing group of the substrate and relatively low reactivity of the catalyst (Table 2 , entry 3). The reactivity improved when we used Pfaltz’s modified Ir catalyst bearing a non-coordinating counter anion (i.e. BAr F ) [44] , [45] , [46] , although this catalyst only afforded the trans isomer (Table 2 , entry 4). The selectivity of this reaction was attributed to intermediate Y2 , where the PMB ether would act as a better directing group rather than the corresponding TIPS ether (Fig. 4b ). Allyl alcohol 5 was therefore used for this conversion. The reaction of 5 under the same conditions [44] , [45] gave aldehyde 4 and alcohol 16b as 2.7:1 isomeric mixtures, respectively (Table 2 , entry 5). This selectivity can be explained by the preferential formation of reaction intermediate Z1 over Z2 , which would suffer considerable steric hindrance (Fig. 4c ). The diastereomeric ratio improved considerably when we used Pfaltz’s modified Ir catalyst to promote the coordination of the substrate to the catalyst, affording an all- cis : trans ratio of 10:1 (Table 2 , entry 6). Most notably, the selectivity of this step was found to be highly reproducible, allowing us to generate gram-scale quantities of the all- cis -substituted cyclopropane 4 for further transformations. Table 2 Formation of all- cis -substituted cyclopropane Full size table Fig. 4 Stereoselectivity of Ir-catalysed double-bond isomerisation. The stereoselectivity of the double-bond isomerisation could be controlled by the directing group. a The Ir catalyst coordinated preferentially to the alcohol moiety in 13 , resulting in the exclusive formation of the all- cis isomer. b Coordination to the TIPS ether was found to be less favourable than the PMB ether, resulting in the formation of the trans isomer through intermediated Y2 . c After the coordination of the alcohol to the catalyst, the reaction proceeded through intermediate Z1 , which was favoured over Z2 because of steric repulsion Full size image Total synthesis of avenaol Having established a successful route to the all- cis -substituted cyclopropane, we turned our attention to the formation of the C ring. Aldehyde 4 was converted to diol 3 by the introduction of an exo methylene at the α position of the aldehyde, followed by a hydroboration (Fig. 5 ). We subsequently screened a wide range of conditions to allow for the differentiation of the hydroxymethyl group. Surprisingly, the diastereoselective DDQ-mediated intramolecular cyclisation of 3 to give acetal 17 resulted in the formation of the caged compound 18 in ~30% yield as a single isomer (Supplementary Table 1 , entry 1). We envisaged that the selective transformation of 18 to 22 via an oxidative ring cleavage reaction would allow for the two hydroxymethyl groups to be differentiated. Thus, we switched our focus to the unexpected formation of the tetrahydropyran ring. The treatment of this system with Cu(OTf) 2 was found to be ineffective, whilst Zn(OTf) 2 and Sc(OTf) 3 gave the cyclised products 18 and 19 (Supplementary Table 1 , entries 2–4). These results indicated that acidic conditions would be important, and that this transformation would proceed via the secondary cation intermediate A . With this in mind, we investigated the addition of BF 3 ·OEt 2 and p -toluenesulfonic acid (pTsOH) (Supplementary Table 1 , entries 6 and 7). The results revealed that pTsOH gave a best yield, although a large portion of the other hydroxy group also reacted with a by-product derived from PMB group to give mixture of 18 and 19 . The addition of thiophenol (PhSH) was effective for trapping this by-product, allowing for the diastereoselective formation of the desired product 18 as a single product. Interestingly, the ring-opening product was not observed under these conditions, most likely because of the stability of the bisected cyclopropylcarbinyl cation intermediate A , where the π-orbitals of the cation would interact with the sp 2 -like orbitals of the cyclopropane ring [47] , [48] , [49] . Fig. 5 Total synthesis of avenaol ( 1 ). Conditions: a aq. CH 2 O, pyrrolidine, EtCO 2 H, i PrOH, 45 °C, then NaBH 4 , MeOH, 0 °C, 75%; b BH 3 ·THF, then aq. NaOH, aq. H 2 O 2 , 88%; c p- toluenesulfonic acid, PhSH, CH 2 Cl 2 , 88%; d BzCl, Et 3 N, DMAP, CH 2 Cl 2 , 86%; e TFDO, CH 2 Cl 2 , −78 °C, f mesyl chloride, Et 3 N, CH 2 Cl 2 ; g NaCN, 15-crown-5, DMSO, 91% (two steps); h diisobutylaluminium hydride, THF, −20 °C; i aq. NaOH, 100 °C, then 1 M aq. HCl; j p- toluenesulfonic acid, benzene, reflux, 49% (three steps); k OsO 4 , 4-methylmorpholine N -oxide, acetone– t BuOH–H 2 O, 63% (dr 14:1); l TESCl, imidazole, DMF, 76%; m t BuOK, HCO 2 Me, THF; n 5-bromo-3-methylfuran-2-one, K 2 CO 3 , 1-methyl-2-pyrrolidinone, 57% (two steps), dr 1:1; o Dess–Martin periodinane, CH 2 Cl 2 –pyr, 39% (for 28 ) and 36% for (C2′-epi- 28 ); p HF·pyr, THF, 97% (for 1 ), 11% (for C2′ epi- 1 ). Bz Benzoyl, TES triethylsilyl, TFDO methyl(trifluromethyl)dioxirane Full size image The C–H oxidation of the tetrahydropyran ring in 18 was investigated for the construction of compound 22 . The alcohol moiety in compound 18 was initially protected by a benzoyl group. 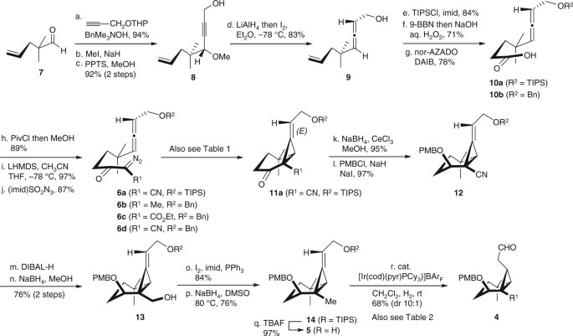Fig. 3 Synthesis of all-cis-substituted cyclopropane4. Conditions: a HC≡CCH2OTHP, BnMe3NOH, DMSO, 94%; b NaH, MeI, THF–DMPU; c pyridiniump-toluenesulfonate, MeOH, 92% (two steps); d LiAlH4then I2, Et2O, −78 °C, 83%; e TIPSCl, imidazole, DMF, 84%; f 9-BBN, then aq. NaOH, aq. H2O2, 71%; g nor-AZADO, DAIB, CH2Cl2–pH 7 buffer, 78%; h PivCl,iPr2NEt, then MeOH, DMAP, 89%; i lithium bis(trimethylsilyl)amide, CH3CN, THF, −78 °C, 97%; j (imidazoyl)SO2N3, pyridine, CH3CN, 87%; k NaBH4, CeCl3, MeOH 95%, (dr 17:1); l PMBCl, NaH, NaI, THF, 0–50 °C, 97%; m diisobutylaluminium hydride, toluene–THF, −78 °C to rt; n NaBH4, MeOH, 0 °C, 76% (two steps); o I2, PPh3, imidazole, CH2Cl2, 0 °C; 84%, p NaBH4, DMSO, 80 °C, 76%; q TBAF, THF, 97%; r [Ir(cod)(pyr)PCy3]BArF, CH2Cl2, H2, 68% (dr 10:1). THP tetrahydropyranyl, DMPUN,N′-dimethylpropylene urea, triisopropylsilyl, DAIB (diacetoxyiodo)benzene, DMAP 4-dimethylaminopyridine,BArF(3,5-bisCF3C6H3)4B− The addition of a stoichiometric charge of CrO 3 or a combination of RuCl 3 and NaIO 4 resulted in the oxidation of the ring to give the undesired lactone 23 and carboxylic acid 24 , respectively (Table 3 , entries 1 and 2). We also conducted the C–H oxidation according to the procedure reported by White’s group using (2 S ,2′ S -(−)-[ N , N ′-bis(2-pyridylmethyl)]-2,2′-bipyrrolidinebis(acetonitrile)iron(II) hexafluoroantimonate (( S , S )-Fe(pdp)) [50] , which gave the desired alcohol 22 in 65% yield via 21 . It is noteworthy, however, that this reaction required a stoichiometric amount of an iron reagent (Table 3 , entry 3). In an attempt to improve the yield, we investigated the use of dimethyldioxirane (DMDO) and methyltrifluromethyldioxirane (TFDO) [51] . The use of an excess of DMDO resulted in a slow reaction (i.e. starting material remaining after 1 day) (Table 3 , entry 4), whereas the use of TFDO at 0 °C gave a mixture of alcohol 22 and lactone 23 , presumably because of its high reactivity (Table 3 , entry 5). This reaction was subsequently performed at −78 °C to improve the regioselectivity and proceeded smoothly to give 22 in excellent yield (Table 3 , entry 6). 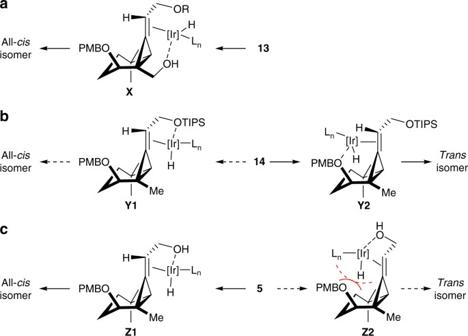Fig. 4 Stereoselectivity of Ir-catalysed double-bond isomerisation. The stereoselectivity of the double-bond isomerisation could be controlled by the directing group.aThe Ir catalyst coordinated preferentially to the alcohol moiety in13, resulting in the exclusive formation of the all-cisisomer.bCoordination to the TIPS ether was found to be less favourable than the PMB ether, resulting in the formation of thetransisomer through intermediatedY2.cAfter the coordination of the alcohol to the catalyst, the reaction proceeded through intermediateZ1, which was favoured overZ2because of steric repulsion Table 3 C–H oxidation of tetrahydrofuran 20 Full size table The final stage of the total synthesis involved the formation of an α-hydroxyketone and the introduction of the D ring of avenaol. Mesylation of the alcohol moiety in 22 , followed by the substitution of the resulting mesylate with cyanide gave the corresponding nitrile (Fig. 5 ). The subsequent reduction of the ketone moiety, hydrolysis of the nitrile and benzoyl protecting groups, followed by an acidic treatment, resulted in the formation of the lactone ring to give 25 . To avoid the possibility of an intramolecular cyclisation between the α position of the lactone and the C2 position of the A ring (Supplementary Fig. 5 ), we proceeded via the dehydration of the alcohol rather than an oxidative transformation. The stereoselective dihydroxylation of 2 , followed by the selective protection of the alcohol at the C3, gave 26 with excellent selectivity. Formylation, followed by the introduction of a butenolide unit 27 [16] gave a mixture of C2′ epimers. Dess–Martin oxidation gave the protected avenaol 28 , which was separated from the corresponding C2′ epi- 28 by column chromatography over silica gel. To determine the stereochemistry, the silyl groups in both 28 and C2′ epi- 28 were subsequently removed using HF·pyridine to give avenaol ( 1 ) and C2′ epi- 1 , respectively. Despite the low yield for the latter of these two reactions, we were able to obtained a crystal of C2′ epi- 1 for X-ray crystallography. 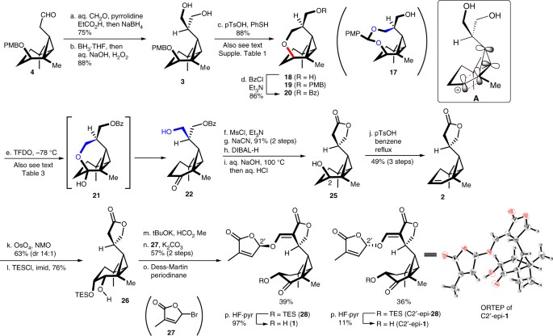Fig. 5 Total synthesis of avenaol (1). Conditions: a aq. CH2O, pyrrolidine, EtCO2H,iPrOH, 45 °C, then NaBH4, MeOH, 0 °C, 75%; b BH3·THF, then aq. NaOH, aq. H2O2, 88%; cp-toluenesulfonic acid, PhSH, CH2Cl2, 88%; d BzCl, Et3N, DMAP, CH2Cl2, 86%; e TFDO, CH2Cl2, −78 °C, f mesyl chloride, Et3N, CH2Cl2; g NaCN, 15-crown-5, DMSO, 91% (two steps); h diisobutylaluminium hydride, THF, −20 °C; i aq. NaOH, 100 °C, then 1 M aq. HCl; jp-toluenesulfonic acid, benzene, reflux, 49% (three steps); k OsO4, 4-methylmorpholineN-oxide, acetone–tBuOH–H2O, 63% (dr 14:1); l TESCl, imidazole, DMF, 76%; mtBuOK, HCO2Me, THF; n 5-bromo-3-methylfuran-2-one, K2CO3, 1-methyl-2-pyrrolidinone, 57% (two steps), dr 1:1; o Dess–Martin periodinane, CH2Cl2–pyr, 39% (for28) and 36% for (C2′-epi-28); p HF·pyr, THF, 97% (for1), 11% (for C2′ epi-1). Bz Benzoyl, TES triethylsilyl, TFDO methyl(trifluromethyl)dioxirane The X-ray crystal structure of C2′ epi- 1 confirmed that the relative stereochemistry between C2′ and C8 was as shown in Fig 5 . Moreover, the spectroscopic data obtained for synthetic avenaol ( 1 ) (i.e. 1 H, 13 C NMR and HRMS) were identical to those of the natural sample 1 [9] . These results therefore confirm that the proposed structure is correct. In summary, we have achieved the total synthesis of avenaol. The key feature of this synthesis is the use of an alkylidenecyclopropane, which allowed for the robust formation of an all- cis -substituted structure via a stereoselective double-bond isomerisation and avoided the cleavage of the cyclopropane ring and the formation of a caged structure. The regioselective formation and C–H oxidation of a tetrahydrofuran ring were also important steps in this synthesis. The interesting structural features of avenaol, including its all- cis -substituted cyclopropane were confirmed to be correct as a consequence of our total synthesis. This established route has provided synthetic samples for further biological evaluation and is also suitable for the synthesis of a range of analogues. Furthermore, this strategy will provide a platform for the synthesis of other natural products containing this structure. The extension of this strategy to structurally related natural products, as well as structure–activity relationship studies of avenaol, are currently underway. General All non-aqueous reactions were run in dried glassware under a positive pressure of argon atomosphere. Reactions were monitored by thin-layer chromatography using Silica gel 60 plates (Merck, Darmstadt, Germany). Silica gel column chromatography was performed using Chromatorex BW-300 (Fuji silysia, Aichi, Japan) and Kanto silica gel 60 (particle size 63–210 μm, Kanto, Tokyo, Japan). Proton nuclear magnetic resonance ( 1 H NMR) spectra were taken with a JNM-AL 400 (JEOL) at 400 MHz or a JNM-ECA 500 (JEOL, Tokyo, Japan) at 500 MHz. Chemical shifts were measured relative to the residual solvent peak in C 6 D 6 ( δ 7.16) or Me 4 Si ( δ 0.00) in CDCl 3 . Multiplicity was indicated by one or more of the following: s (singlet); d (doublet); t (triplet); q (quartet); m (multiplet); br (broad). Carbon nuclear magnetic resonance ( 13 C NMR) spectra were recorded on a JNM-AL 400 at 100 MHz or a JNM-ECA 500 at 126 MHz. Chemical shifts were measured relative to CDCl 3 ( δ 77.0) or C 6 D 6 ( δ 128). Infrared spectra were collected on a FT/IR-4100 Fourier-transform infrared spectrometer (JASCO, Tokyo, Japan) as ATR (attenuated total reflectance). Low and high-resolution mass spectra were recorded on a LCMS-IT-TOF (Shimadzu, Kyoto, Japan) for ESI-MS and JMS-700 mass spectrometer (JEOL) for FAB-MS. Experimental data For the experimental procedures and spectroscopic and physical data of the compounds and the crystallographic data of C2′-epi avenaol, see Supplementary Methods . For NMR spectra of synthetic intermediates, see Supplementary Figs. 5 – 35 . For the comparisons of 1 H and 13 C NMR spectra of the natural and synthetic avenaol, see Supplementary Figs. 36 and 37 . Data availability The X-ray crystallographic coordinates for the structure of C2′-epi avenaol have been deposited at the Cambridge Crystallographic Data Centre (CCDC), under deposition number 1544731. These data can be obtained free of charge from The Cambridge Crystallographic Data Centre via www.ccdc.cam.ac.uk/data_request/cif . Other data are available from the authors upon reasonable request.